Ultrathin and lightweight organic solar cells with high flexibility Application-specific requirements for future lighting, displays and photovoltaics will include large-area, low-weight and mechanical resilience for dual-purpose uses such as electronic skin, textiles and surface conforming foils. Here we demonstrate polymer-based photovoltaic devices on plastic foil substrates less than 2 μm thick, with equal power conversion efficiency to their glass-based counterparts. They can reversibly withstand extreme mechanical deformation and have unprecedented solar cell-specific weight. Instead of a single bend, we form a random network of folds within the device area. The processing methods are standard, so the same weight and flexibility should be achievable in light emitting diodes, capacitors and transistors to fully realize ultrathin organic electronics. These ultrathin organic solar cells are over ten times thinner, lighter and more flexible than any other solar cell of any technology to date. Lightweight and mechanically resilient solar power sources are of increasing interest for modern applications such as electronic textiles, synthetic skin and robotics [1] , [2] . Organic photovoltaic (OPV) solar cells are highly promising in this sector. The thin-film devices comprise two electrodes, a light-harvesting active layer and blocking or transport layers. The total thickness of a functional OPV cell is only a few hundred nanometres. Primary benefits of OPV cells are often listed as low cost, low weight, flexibility and compatibility with reel-to-reel processing for high volume production [3] , [4] . Efficiency and lifetime have reached commercially acceptable levels and flexible modules with roughly 1.5% power conversion efficiency, and over 1 year lifetimes are already on the market [5] . Mitsubishi Chemical Holdings have attained laboratory-scale cell efficiencies of 10% [6] . Weight and flexibility are two of the primary benefits of OPV; yet these mechanical properties are entirely dominated by the device substrate, which leaves much room for advancement of this technology. Among the thinnest reported substrates for OPV devices are 125-μm plastic foils [7] , [8] , [9] . The resulting solar cells are highly flexible with a radius of curvature of 5 mm. It is further interesting to consider not only flexibility but also stretchability. Stretchable inorganic PV devices were made from an array of GaAs microcells arranged in a sub-module configuration with high areal coverage on a patterned polydimethylsiloxane (PDMS) supporting layer. They have demonstrated 20% strain and wrapping around cylinders with 1.5 mm radius [10] . Stretchable organic solar cells have been fabricated directly on pre-stretched PDMS (thickness 200–500 μm), which can then attain 27% tensile strain reversibly [11] . A liquid metal back contact was used to improve mechanical stability. For both the stretchable and flexible OPV devices, the actual solar cell still constitutes <0.25% of the total device thickness. In this work, we answer the questions 'how light?' and 'how flexible?' OPV can be by demonstrating the extremes achievable today. We present ultrathin, light, flexible and compliant OPV devices constructed on only 1.4-μm-thick polyethylene terephthalate (PET) substrates, where the total thickness of the device is less than a typical thread of spider silk. The substrate is commercially available Mylar 1.4 CW02, a commodity scale PET film commonly used as a foil capacitor dielectric. We obtain solar cells with 4.2% power conversion efficiency, an unprecedented specific weight value of 10 W g −1 , high flexibility and can reversibly attain tensile strains of more than 300% on an elastomeric support. Ultrathin solar cells An ultrathin OPV cell is shown schematically in Fig. 1a . Note that the thickness of each layer is drawn to scale. The total device is only 1.9 μm thick, where about one-quarter of the thickness is the active solar cell. Apart from the substrate, all of the materials used for our devices are well established materials for OPV, including poly(3,4-ethylenedioxythiophene):poly(styrenesulphonate) (PEDOT:PSS), poly(3-hexylthiophene) (P3HT), (6,6)-phenyl-C 61 -butyric acid methyl ester (PCBM) and Ca/Ag evaporated metal electrodes. Using these materials, OPV devices on indium tin oxide (ITO)-coated glass substrates have been certified with efficiency up to 4.3% [12] . Using the ITO-free architecture on PET, we obtain comparable efficiency while demonstrating the extreme mechanical properties of organic solar cells. 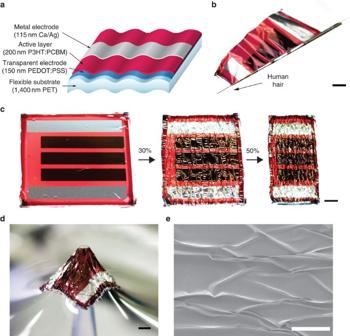Figure 1: Sub-2-μm-thick organic solar cells. (a) Scheme of the ultra-light and flexible organic solar cell. The layer thicknesses are drawn to scale. (b) Extreme bending flexibility demonstrated by wrapping a solar cell around a 35-μm-radius human hair. Scale bar (also inc,d) 2 mm. (c) Stretchable solar cells made by attaching the ultrathin solar cell to a pre-stretched elastomer. They are shown flat (left) and at 30% (middle) and 50% (right) quasi-linear compression. (d) The device attached to the elastomeric support, under three-dimensional deformation by pressure from a 1.5 mm-diameter plastic tube. (e) SEM image of the PET surface of the solar cell in compressed state. The radius of curvature for the shown wrinkles is estimated to be on the order of 10 μm. Scale bar 500 μm. Figure 1: Sub-2-μm-thick organic solar cells. ( a ) Scheme of the ultra-light and flexible organic solar cell. The layer thicknesses are drawn to scale. ( b ) Extreme bending flexibility demonstrated by wrapping a solar cell around a 35-μm-radius human hair. Scale bar (also in c , d ) 2 mm. ( c ) Stretchable solar cells made by attaching the ultrathin solar cell to a pre-stretched elastomer. They are shown flat (left) and at 30% (middle) and 50% (right) quasi-linear compression. ( d ) The device attached to the elastomeric support, under three-dimensional deformation by pressure from a 1.5 mm-diameter plastic tube. ( e ) SEM image of the PET surface of the solar cell in compressed state. The radius of curvature for the shown wrinkles is estimated to be on the order of 10 μm. Scale bar 500 μm. Full size image The P3HT:PCBM bulk heterojunction solar cell is fabricated on a PEDOT:PSS-coated 1.4-μm-thick PET substrate foil. The top electrode is 115 nm Ca/Ag. Figure 1b illustrates the extreme bending flexibility of the solar cell, wrapped around a human hair with a radius of 35 μm. Figure 1c (left) depicts a solar cell on a 100-μm-thick pre-stretched 3 M VHB 4905 elastomer. As the compressive strain of the elastomer is increased to 30% and then 50%, it is evident that the solar cell becomes wrinkled. This enables the solar cell to be stretched back to the pre-strain defined by the elastomer. In standard notation, 50% compressive strain corresponds to 100% tensile strain from the wrinkled reference state. Pictures of a device undergoing a sequence of stepwise compression and re-stretching are shown in Supplementary Fig. S1 . The extreme conformability of an ultrathin organic solar cell is demonstrated by deforming the cell on an elastomeric substrate with a plastic tube of 1.5 mm tip diameter in Fig. 1d . The scanning electron microscopy (SEM) image of the compressed solar cell in Fig. 1e highlights the random network of wrinkles with extremely small bending radii. The ultrathin flexible substrate is available on rolls in large area for industrial use. It is completely compatible with reel-to-reel processing and, therefore, is advantageous for high throughput fabrication. Supplementary Table S1 contains more details on the material properties of the substrate. An atomic force microscopy (AFM) topography image of the PET foil shown in Fig. 2 (left) reveals a root mean square (RMS) surface roughness of ≈12 nm and a maximum height of 162 nm for randomly distributed peaks. AFM images of the subsequent PEDOT:PSS (centre) and P3HT:PCBM (right) layers on the PET show similar RMS roughness of 12 and 16 nm, respectively, and peak heights of 116 and 130 nm. This substrate is very rough compared with the nominal PEDOT and P3HT film thicknesses of 150–200 nm. However, the roughness does not negatively affect the performance of the solar cells. 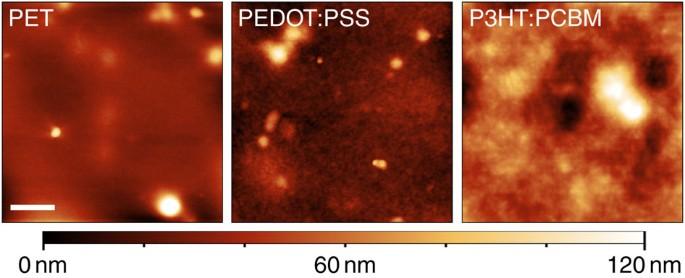Figure 2: AFM images of the individual device layers. AFM topographical image of the 1.4 μm Mylar CW02 substrate foil on glass/PDMS support (left). The RMS roughness is ≈12 nm with a maximum peak-to-peak distance of 162 nm. Image of the PEDOT:PSS transparent electrode on PET (centre). RMS roughness is ≈12 nm and the maximum peak-to-peak distance is 116 nm. Image of the P3HT:PCBM active layer atop the transparent electrode (right). The RMS roughness is ≈16 nm and the maximum peak-to-peak distance is 130 nm. Scale bar 1 μm. Figure 2: AFM images of the individual device layers. AFM topographical image of the 1.4 μm Mylar CW02 substrate foil on glass/PDMS support (left). The RMS roughness is ≈12 nm with a maximum peak-to-peak distance of 162 nm. Image of the PEDOT:PSS transparent electrode on PET (centre). RMS roughness is ≈12 nm and the maximum peak-to-peak distance is 116 nm. Image of the P3HT:PCBM active layer atop the transparent electrode (right). The RMS roughness is ≈16 nm and the maximum peak-to-peak distance is 130 nm. Scale bar 1 μm. Full size image In order to facilitate laboratory-scale device construction, the substrate is cut to size and placed onto a supporting glass plate. The PET adheres to the PDMS-coated glass via weak van der Waals bonding, which allows standard laboratory processes such as spin coating, thermal annealing and vacuum evaporation. The primary functions of the glass support are to maintain planarity during processing and to ease the handling of the device, and the PET can be easily removed by peeling it away. Exact processing details are found in the Methods section. Solar cell efficiency Before removing the solar cell from the supporting glass, the device J – V characteristics are measured under a solar simulator (approximately the A.M. 1.5 Global spectrum with 100 mW cm −2 intensity and spectral mismatch correction), and in the dark. After removal from the supporting glass, it is difficult to maintain planarity in the device, and therefore to know the incident area for calculation of current density ( J ) and power conversion efficiency ( η ). All measurements while the device is still attached to the glass support are scaled per unit area, using a conservative area estimate as the PEDOT:PSS transparent electrode is difficult to pattern exactly. The data reported in subsequent sections, for mechanical stretching and cycling, are not scaled to area and only total current and power are reported for comparison during mechanical manipulation. The J – V characteristics of an optimized ultrathin OPV device are shown in Fig. 3a . This particular device performs with open circuit potential ( V OC )=580 mV, short circuit current ( J SC )=11.9 mA cm −2 , fill factor (FF)=61% and η =4.2% under one sun illumination. This is a representative sample from over 50 devices constructed with various parameters. The average device performance metrics for the nominally identical optimized devices are η =3.9±0.3%, V OC =570±15 mV, J SC =11.3±0.7 mA cm −2 and FF=59±3%. 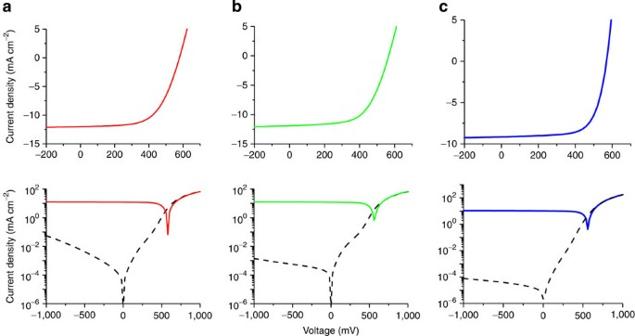Figure 3:J–Vcharacteristics. (a) Linear–linear (top) and log-linear (bottom)J–Vcharacteristics of an optimized ultrathin OPV device on 1.4 μm PET substrate. The device performance metrics areVOC=580 mV,JSC=11.9 mA cm−2, FF=61% andη=4.2%. Solid lines are measured under one sun illumination and dashed lines in the dark (also inb,c). (b) Device performance of reference device, using the same materials but constructed directly on glass substrates without PET. The device performance metrics areVOC=565 mV,JSC=11.9 mA cm−2, FF=61% andη=4.1%. Comparing theJ–Vcurves ofaandb, nearly identical behaviour is observed. TheVOCof this particular device is slightly lower, but overall the performance of the glass and PET-based solar cells is indistinguishable. (c) Ultrathin OPV devices on PET foil with underlying silver grid can attain FF up to 71% (top) and dark diode rectification of up to 6 orders of magnitude at ±1 V (bottom). However, they typically show lowerJSCdue to shading from the silver grid. Figure 3: J – V characteristics. ( a ) Linear–linear (top) and log-linear (bottom) J – V characteristics of an optimized ultrathin OPV device on 1.4 μm PET substrate. The device performance metrics are V OC =580 mV, J SC =11.9 mA cm −2 , FF=61% and η =4.2%. Solid lines are measured under one sun illumination and dashed lines in the dark (also in b , c ). ( b ) Device performance of reference device, using the same materials but constructed directly on glass substrates without PET. The device performance metrics are V OC =565 mV, J SC =11.9 mA cm −2 , FF=61% and η =4.1%. Comparing the J – V curves of a and b , nearly identical behaviour is observed. The V OC of this particular device is slightly lower, but overall the performance of the glass and PET-based solar cells is indistinguishable. ( c ) Ultrathin OPV devices on PET foil with underlying silver grid can attain FF up to 71% (top) and dark diode rectification of up to 6 orders of magnitude at ±1 V (bottom). However, they typically show lower J SC due to shading from the silver grid. Full size image These results are comparable to leading BHJ OPV devices using P3HT:PCBM on ITO-coated glass substrates [12] . The scarcity and cost of indium, and the requirement of smooth substrates for thin films are considered to be significant hurdles for mass production of OPV devices [13] , [14] . The surface roughness of the PET substrate, and the high-conductivity PEDOT:PSS in place of ITO do not significantly reduce the device efficiency. Devices fabricated on the ultrathin PET substrate show nearly the same performance metrics as nominally identical reference samples prepared on glass substrates. Representative J – V curves for devices on glass substrates are shown in Fig. 3b . Of primary concern are the transparency and conductivity of the PEDOT:PSS transparent electrode. By varying the thickness of the layer, there is a trade-off between FF and J SC , as a thicker electrode will be more conductive but less transparent. One of the best-performing devices is shown in Fig. 3a . However, through mass construction of the devices with slight variations, we have obtained a wide range of FF (up to 71%) and J SC (up to 12 mA cm −2 ) though not in the same device. Devices with an additional silver grid underlying the PEDOT:PSS electrode are shown in Fig. 3c . They exhibit FF up to 71% due to a lowered serial resistance, but without thorough optimization, a reduced J SC is found. For small, laboratory-scale devices the silver grid is unnecessary and detrimental to device performance, but it will doubtlessly be required for large-area devices. Diodes with a dark rectification of up to 6 orders of magnitude were obtained, though they did not show a high efficiency. Extreme mechanical deformation The primary goal in constructing such thin devices is to demonstrate continuous optoelectronic operation under extreme mechanical deformation. In order to do so, we transfer the device from the glass support to a pre-stretched elastomer (3 M VHB 4905). The device on PET sticks to the elastomer very well, and the glass support can be removed. Two rigid plastic spacers are placed on the elastomer, leaving a gap of 1 cm for the compression and stretching of the device. This assures that the strain will be nearly one dimensional and concentrated in the region of the active device, which occupies roughly half of the 1 cm gap. The rigid spacers are brought closer together in steps of 1 mm, corresponding to 10% compression. For each step, the I - V characteristics are measured under the solar simulator, and the results are shown in Fig. 4a . It is clear that the device remains a functional solar cell down to 80% compression. Upon re-stretching the device, it returns to its pre-compression operation state. According to accepted definitions for stretchable conducting films, this re-stretching process corresponds to 400% tensile strain in a fully functional solar cell, where 300% is considered ultrahigh for a single conducting film [15] . A more detailed description of the calculation of compression and tensile strain is given in the Methods section, and an illustration of the compression/stretching apparatus is shown in Supplementary Fig. S2 . The V OC , I SC , FF and output power are plotted as a function of compression (and corresponding tensile strain) in Fig. 4b , all normalized to their pre-compression value. As the incident area should track linearly with the compression, we would expect the I SC and power to scale exactly with the compression, following the black line in Fig. 4b . We can see that both values are consistently higher than the device area scaling. 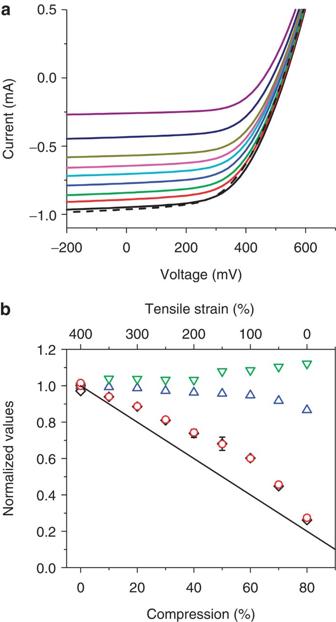Figure 4: Extreme mechanical deformation. (a)I-Vcurves during compression on pre-stretched elastomer. The solid black line represents 0% and the purple line represents 80% compression with the intermediate steps of 10% distributed between accordingly. The dashed black line represents the device after re-stretching from 80% compression to its initial flat state. (b) Measured device parameters 0–80% compression, which correspond to 400–0% tensile strain or five times change in size. Green downward triangles represent FF, blue upward trianglesVOC, red circlesISCand black diamonds power. All parameters are normalized to their pre-compression value. TheISCand correspondingly the total maximum power of the solar cell decrease, but maintain higher values than would be expected with the corresponding decrease of device area, represented by the black line. Upon re-stretching the device to its original size, the values are nearly identical to the pre-compression state. The symbol size is chosen to represent the reproducibility of the experiment, as indicated by error bars for selected data points for the power metric. Figure 4: Extreme mechanical deformation. ( a ) I-V curves during compression on pre-stretched elastomer. The solid black line represents 0% and the purple line represents 80% compression with the intermediate steps of 10% distributed between accordingly. The dashed black line represents the device after re-stretching from 80% compression to its initial flat state. ( b ) Measured device parameters 0–80% compression, which correspond to 400–0% tensile strain or five times change in size. Green downward triangles represent FF, blue upward triangles V OC , red circles I SC and black diamonds power. All parameters are normalized to their pre-compression value. The I SC and correspondingly the total maximum power of the solar cell decrease, but maintain higher values than would be expected with the corresponding decrease of device area, represented by the black line. Upon re-stretching the device to its original size, the values are nearly identical to the pre-compression state. The symbol size is chosen to represent the reproducibility of the experiment, as indicated by error bars for selected data points for the power metric. Full size image The optimistic explanation for this would be an enhancement in light harvesting due to micro-texturing upon folding the device. In the compressed state, there is more light absorbing polymer per unit incident area. Light not absorbed on the first pass through the active layer could also be reflected back into the device on the other side of a crease, allowing for improved overall absorption. This is evident in the relative total reflectance of the sample shown in Supplementary Fig. S3 , where less light is reflected in various stages of compression. Additionally, the compression does not decrease the device area uniformly. As the device area is defined by the metal back electrode, it is likely that the overall substrate compresses more on the edge. Thus, when the total compression is 50%, the device area is not reduced by exactly the same value. This effect can be seen in Supplementary Fig. S1 , upon the very first compression of the sample. It becomes much less prominent on the subsequent cycles. Compression values greater than 60% likely approach the limit of the test fixture, and the physical deformation may no longer be quasi-linear. There is evidence for both an increase in light harvesting and an error in area estimation upon compression. The complex formation of folds and wrinkles, as seen in Fig. 1 and Supplementary Fig. S1 , also allows biaxial compression. In order to attach the solar cell to the elastomer, now pre-stretched in two directions, the rigid plastic pieces that constricted the compression to one dimension were left off. This makes the actual compression of the device much less certain. Device performance under reversible biaxial compression is shown in Fig. 5a , where the device withstands roughly 20% biaxial compression and re-stretching. The device stays functional even at very high biaxial compression of more than 50% ( Fig. 5b ). I SC and power output scale roughly proportional to a decrease in area. The overall biaxial stretch behaviour is similar to the uniaxial stretch described above. 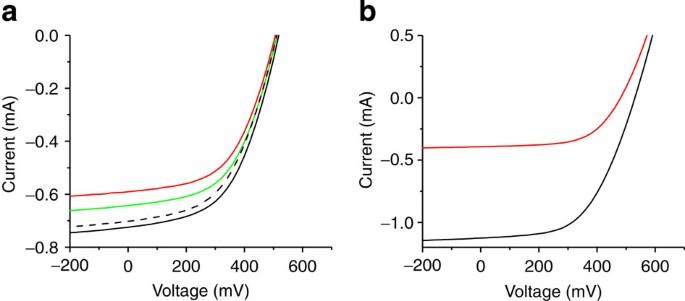Figure 5: Biaxial compression. (a) The device performance under reversible biaxial compression of 0% (black solid line), roughly 10% (green solid line) and roughly 20% (red solid line). Upon re-stretching to near flat conditions, the device shows comparable performance (black dashed line). (b) Device performance under very high biaxial compression of more than 50% (red solid line) compared with 0% flat state (black solid line). Figure 5: Biaxial compression. ( a ) The device performance under reversible biaxial compression of 0% (black solid line), roughly 10% (green solid line) and roughly 20% (red solid line). Upon re-stretching to near flat conditions, the device shows comparable performance (black dashed line). ( b ) Device performance under very high biaxial compression of more than 50% (red solid line) compared with 0% flat state (black solid line). Full size image This approach for stretchable solar cells has several distinct advantages. The fabrication processes used are entirely planar, avoiding transfer printing processes, and are thus reel-to-reel compatible. Any microstructuring, surface conformation or other physical manipulation can be performed subsequently, without integrating specific geometries into cell construction. Adhesion to a pre-streched elastomer is done in a single step after device fabrication. The complete solar cells show large, reversible quasi-linear compression ratios over 70%, corresponding to a tensile strain of more than 300% from the wrinkled state. Cyclic stretching Though compression and stretching of the device induces very little change in the device performance, there may be small changes that accumulate over many cycles. To investigate the durability of the devices under repeated stretching and compression, we cycled the device from 0% (original size) to 50% quasi-linear compression and back more than 20 times. At each cycle the I-V characteristics were measured under the solar simulator, both in the compressed and extended state. The cycling test showed a gradual decrease in the I SC , the FF and the output power, resulting in a 27% decrease in power after 22 cycles. The I-V curves at 0 and 50% compression for selected cycles are shown in Fig. 6a, and the normalized device parameters at each full (extended) cycle are shown in Fig. 6b . 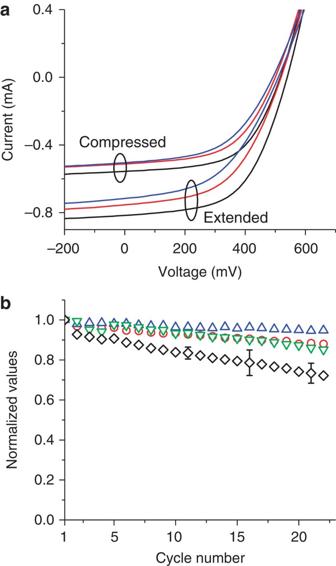Figure 6: Resilience to cyclic compression–stretching. Device performance during 22 consecutive compression–stretch cycles to 50% compression. (a) TheI-Vcharacteristics are shown at 1 (black), 11 (red) and 22 (blue) cycles for both the fully extended and 50% (quasi-linear) compressed states. (b) Device performance metrics plotted at each of the 22 cycles for the fully extended state. Green downward triangles represent FF, blue upward trianglesVOC, red circlesISCand black diamonds power. All parameters are normalized to their initial value. Upon cycling, a reduction of the FF andISCis observed. The origin of these losses is unknown, but is certainly in part owing to the experimental apparatus and loss of contact. The overall efficiency is shown to be 73% of its original value after 22 repeated cycles. Multiple separate devices were subjected to cyclic testing. For the sake of clarity, error bars are indicated only for the power metric for selected data points, as this is the primary metric for device characterization. Figure 6: Resilience to cyclic compression–stretching. Device performance during 22 consecutive compression–stretch cycles to 50% compression. ( a ) The I-V characteristics are shown at 1 (black), 11 (red) and 22 (blue) cycles for both the fully extended and 50% (quasi-linear) compressed states. ( b ) Device performance metrics plotted at each of the 22 cycles for the fully extended state. Green downward triangles represent FF, blue upward triangles V OC , red circles I SC and black diamonds power. All parameters are normalized to their initial value. Upon cycling, a reduction of the FF and I SC is observed. The origin of these losses is unknown, but is certainly in part owing to the experimental apparatus and loss of contact. The overall efficiency is shown to be 73% of its original value after 22 repeated cycles. Multiple separate devices were subjected to cyclic testing. For the sake of clarity, error bars are indicated only for the power metric for selected data points, as this is the primary metric for device characterization. Full size image There are several possible reasons for the device degradation during this measurement. We suspect that the I SC decreases gradually because the device never fully returns to its original incident area. The elastomer is visco-elastic and therefore permanently deforms over time. This is evident after cycling, as there are still visible ripples in the device. The reduction in FF may be due to increased resistivity of the metal or PEDOT:PSS electrodes. Both layers may form cracks under repeated cycling, which reduces the conductivity and increases the series resistance of the device [16] . However, cyclic tests of resistivity of Ag and PEDOT:PSS layers on the same PET substrate are shown in Supplementary Fig. S4 . The resistance increases by <10% in a Ag film and there is no detectable increase seen in PEDOT:PSS after 100 cycles. There is also an additional resistance induced by the deterioration of the rigid metal wire contact. It is difficult to quantify the contributions from the external contact and the actual device degradation. But in all of our tests, the external wire broke loose before the device degraded catastrophically. The power conversion efficiency of a solar cell corresponds directly to the power per unit area, and is the primary metric for describing solar cell performance. However, area is not always the limiting parameter. When considering solar power for certain applications, the power output per weight (specific weight in Watts per gram) may be a more appropriate metric. This is particularly true for situations that require portable power, where payload is a premium such as aircraft, spacecraft or personal pack load. The specific weight of various solar technologies (panels and cells) for terrestrial and space applications is compared in Fig. 7 . Commercially available space-rated high-efficiency Si and triple junction cells have 0.82 and 0.39 W g −1 , respectively [17] . A recent report showed that CIGS cells were constructed on thin (25 μm) polyimide films with 18.7% efficiency [18] . These devices have an extremely high specific weight of roughly 3 W g −1 . The OPV devices constructed on PET presented here have a per-area mass of 4 g m −2 , and 4% efficiency, giving 10 W g −1 . 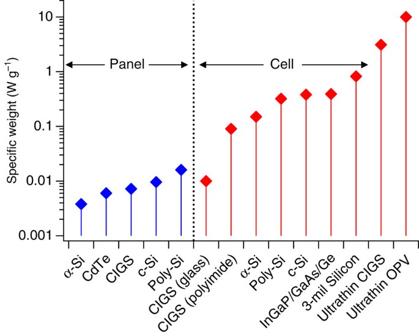Figure 7: Comparing solar cell technologies. Specific weight of various photovoltaic technologies for complete modules (left) and individual cells (right). Module data are taken from manufacturer-specified efficiency and weight of commercially available panels and should be representative: Kaneka 12V 55W PV Module, First Solar FS272, Sunforce 70W Pro Series, Bosch Solar Module c-Si M60 and Kyocera KD245Gx-LPB. Cell data were taken from published academic results. In many cases, the cell weight was not published and so was estimated from published layer thicknesses and known material densities, assuming 2% areal coverage for metal grid contacts17,18,23,24,25,26,27. For a direct comparison of cell efficiency, please see Greenet al6. Figure 7: Comparing solar cell technologies. Specific weight of various photovoltaic technologies for complete modules (left) and individual cells (right). Module data are taken from manufacturer-specified efficiency and weight of commercially available panels and should be representative: Kaneka 12V 55W PV Module, First Solar FS272, Sunforce 70W Pro Series, Bosch Solar Module c-Si M60 and Kyocera KD245Gx-LPB. Cell data were taken from published academic results. In many cases, the cell weight was not published and so was estimated from published layer thicknesses and known material densities, assuming 2% areal coverage for metal grid contacts [17] , [18] , [23] , [24] , [25] , [26] , [27] . For a direct comparison of cell efficiency, please see Green et al [6] . Full size image This extreme specific weight may be advantageous for certain applications. Weather balloons, unmanned aircraft or any other remote sensing systems may prioritize specific weight and have known project duration. The same is true for pack-weight for remote wilderness use, where there is often a need for lightweight power sources. Modern robotics applications, such as electroadhesive wall climbing and at-scale robotic insects, have very specific needs for low-weight power [19] , [20] . Ultrathin OPV may be ideal for such applications. These particular materials are not comparable to the most efficient or air-stable organic semiconductors, inter-layers or electrodes used in state-of-the-art OPV devices [6] , [21] ; so there is a large potential for optimization by enhancing both efficiency and lifetime of such ultrathin OPV devices while maintaining low weight and high flexibility. In conclusion, polymer-based solar cells have been constructed on 1.4-μm-thick PET substrate. The devices use standard OPV materials and obtain nearly identical efficiency to those constructed on ITO-coated glass substrates with over 4% power conversion efficiency. Here, the high conductivity PEDOT:PSS electrode replaces the ITO, which is considered a cost- and production-volume-limiting material [13] . The polymer electrode is highly flexible compared with the ternary oxide [22] . The device layers consist of roughly 450 nm total thickness, so the total device including substrate is <2 μm. These ultrathin, flexible solar cells show unprecedented mechanical resilience. By adhering the flexible device to a pre-stretched elastomer, we have shown that the devices survive quasi-linear compression to below 70% of their original area. Furthermore, we have shown cyclic compression and stretching to 50%, over more than 20 full cycles with marginal loss in device performance and no visible defect formation beyond the external contact points. Though the electrically active components of this device are in principle no different than other standard OPV devices, the solar cell now constitutes roughly 25% of the total thickness and 45% of the total weight. OPV is emerging as a viable technology where temporary, high-volume and low-weight power sources are required. The extreme flexibility and specific weight demonstrated here realize the unique potential for OPV as an ultrathin-film power source. Substrate preparation Rigid glass slides, coated with an ≈500-nm-thick PDMS layer, served as supporting substrates for the 1.4-μm-thick PET foils. The PET is Mylar ® 1.4 CW02, obtained from Pütz GMBH + Co. Folien KG. Adhering the PET film to the supports readily enabled all subsequent planar processing steps including spin coating, thermal annealing and vacuum deposition. The devices could be peeled off the supporting stack without causing damage to the solar cells. Device fabrication We spun PEDOT:PSS (Clevios PH1000, with 5 vol% dimethylsulphoxide, and mixed with 0.5. vol% Zonyl FS-300 fluorosurfactant from Fluka to promote wetting on the hydrophobic PET) at 1,000 r.p.m. for 60 s and then 2,000 r.p.m. for 60 s onto the PET films. The samples were dried on a hotplate at 120 °C for 30 min, yielding 150-nm-thick PEDOT:PSS layers with ~100 Ω sq −1 . A solution of 30 mg ml −1 P3HT (obtained from Plextronics and purified by repeated reprecipitation) and 30 mg ml −1 PCBM (from Solenne BV) in dichlorobenzene was spun at 1,500 r.p.m. for 120 s. The P3HT:PCBM was partly wiped away with a toluene-soaked cotton swab, exposing some of the PEDOT:PSS to allow for contacting. P3HT:PCBM films of 200 nm thick were obtained. The samples were transferred to a nitrogen-filled glovebox and annealed on a hotplate at 150 °C for 15 min. Finally, 15 nm Ca and 100 nm Ag were thermally evaporated at 1 Å s −1 and pressure of 10 −6 mbar. Typical devices had an active area of 0.1 cm 2 . Device characterization The devices were first characterized in the dark and under illumination of a solar simulator (A.M. 1.5 Global spectrum with 100 mW cm −2 intensity with spectral mismatch correction). I-V characteristics were recorded using a Keithley 236 source metre. All I-V measurements were carried out in a nitrogen-filled glovebox. Layer thicknesses were measured with a Digital Instruments Dimension 3100 AFM. The s.e.m. images of solar cells atop the elastic substrate were taken after fixing the samples onto a rigid glass substrate and depositing a thin (<20 nm) gold layer with a Hitachi S-4800 Field Emission Scanning Electron Microscope at a acceleration voltage of 20 kV. Compression and stretching A schematic of the compression/stretching apparatus is shown in Supplementary Fig. S2 . We place the 3 M VHB 4905 elastomer between the two clamps and stretch it by moving the clamps further apart. We then place rigid delimiters to define a compression and stretching zone, where the distance between the two rigid delimiters is exactly 1 cm. We define this to be L 0 . Then we place the solar cell onto the elastomer. The active area of the cell is roughly 2×5 mm 2 , and we align the long dimension in the direction of the compression. Thus, the cell occupies roughly half of the 1 cm gap in the compression direction. We then compress the cell by moving the rigid delimiters closer together, allowing the elastomer to relax, which compresses the device area. The compression zone is 5×1 cm 2 , so the deformation is quasi-linear and quasi-reversible, though there is always a small, unintentional bi-axial and/or permanent deformation due to the visco-elasticity of the elastomer. The area changes with the linear change in distance between the rigid delimiters. We define the compression to be ( L 0 − L )/ L 0 . Shrinking the gap from 10 to 2 mm corresponds to an 80% compression. The definition of tensile strain uses the fully relaxed (smallest) state as the starting point. So after relaxing to 2 mm, re-stretching to 10 mm would give a tensile strain of (10–2 mm)/2 mm, or 400% tensile strain. Both 80% compression and 400% tensile strain refer to a five times change in device area, and use either the fully stretched or fully compressed state to normalize. How to cite this article: Kaltenbrunner, M. et al . Ultrathin and lightweight organic solar cells with high flexibility. Nat. Commun. 3:770 doi: 10.1038/ncomms1772 (2012).